Maintenance of protein synthesis reading frame by EF-P and m1G37-tRNA Maintaining the translational reading frame poses difficulty for the ribosome. Slippery mRNA sequences such as CC[C/U]-[C/U], read by isoacceptors of tRNA Pro , are highly prone to +1 frameshift (+1FS) errors. Here we show that +1FS errors occur by two mechanisms, a slow mechanism when tRNA Pro is stalled in the P-site next to an empty A-site and a fast mechanism during translocation of tRNA Pro into the P-site. Suppression of +1FS errors requires the m 1 G37 methylation of tRNA Pro on the 3' side of the anticodon and the translation factor EF-P. Importantly, both m 1 G37 and EF-P show the strongest suppression effect when CC[C/U]-[C/U] are placed at the second codon of a reading frame. This work demonstrates that maintaining the reading frame immediately after the initiation of translation by the ribosome is an essential aspect of protein synthesis. Maintenance of the translational reading frame is an important open question in biology. Loss of the reading frame due to spontaneous +1 frameshift (+1FS) errors is deleterious, resulting in premature termination of gene expression. However, despite the dynamic movement of successive tRNA molecules and associated mRNA from the A-site to the P-site and to the E-site, each ribosome manages to stay in the correct reading frame (0-frame) through hundreds of codons. At a rapid rate of incorporating 10–20 amino acids per second into the nascent chain, an E. coli ribosome makes less than one +1FS error per 30,000 amino acids [1] , a frequency at least tenfold lower relative to other types of translation errors. How is the reading frame maintained so faithfully? Although early genetic work suggested a model of tRNA shifting by quadruplet base pairing, subsequent isolation of non-tRNA suppressors invalidated this model [2] , [3] . More recent work favoured a model of tRNA slippage from a stalled P-site [2] , [3] , although the mechanism that drives the slippage remains unknown. Here we provide molecular-level insights into the speed, frequency and timing of +1-frameshifting and the cellular factors that suppress such errors. Protein synthesis in bacteria begins with the assembly of the large and small ribosomal subunits (50S and 30S) into a 70S initiation complex (70SIC) that places the initiator fMet-tRNA fMet at the AUG start codon at the P-site. Upon accommodation of the in-frame aminoacyl-tRNA at the A-site, the 70SIC synthesizes the first peptide bond and moves the newly synthesized peptidyl-tRNA from the A- to the P-site in the first round of translocation to enter into the elongation phase. Maintaining the reading frame during elongation is most challenging for the ribosome at ‘slippery’ mRNA sequences. Sequences such as CC[C/U]-[C/U] are particularly slippery [4] , because the codon–anticodon interaction with the cognate GGG isoacceptor tRNA Pro , for example, is identical in the 0- and +1-frame, indicating a minimum energetic penalty for the tRNA to shift to the +1-frame. 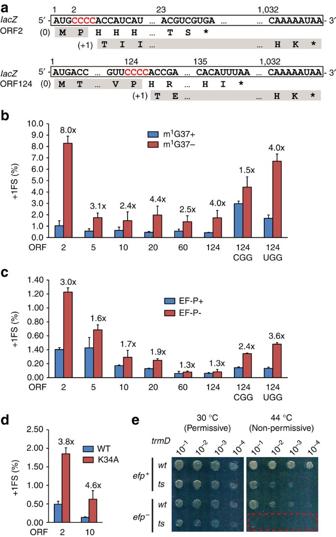Figure 1: Suppression of cellular +1FS errors by m1G37 and EF-P. (a) Suppression of +1FS errors was monitored usinglacZreporter genes containing the CCC-C frameshift site (in red) adjacent to the AUG start codon or further downstream. Examples are shown for the Open Reading Frame (ORF) 2 construct with the CCC-C at the 2nd codon position and the ORF124 construct with the CCC-C at the 124th codon position. Normal translation at each CCC-C site would result in premature termination of β-gal synthesis (indicated by the symbol *) unless a +1FS event occurred with tRNAPro. The +1FS frequency is expressed as the ratio of β-gal of the +1-frame reporter with the CCC-C sequence over the in-frame reporter with the CCC sequence. (b) Measurement of +1FS frequency of each reporter in anE. coli trmD-KOstrain with and without the synthesis of m1G37. ThistrmD-KOstrain was maintained viable by expressing the human counterparttrm5on an arabinose-controlled expression plasmid. The m1G37+ condition was achieved with 0.2% (w/v) arabinose, whereas the m1G37- condition was achieved without arabinose. (c) Measurement of +1FS frequency of each reporter construct in an isogenic pair ofE. coli efp+versusefp−strains. (d) Measurement of +1FS frequency of ORF2 and ORF10 in theE. coli efp−strain complemented by WT or K34A mutant of EF-P co-expressed withyjeAandyjeK. Inb–d, each +1FS frequency is the average of at least three independent measurements, with the errors showing s.d. (standard deviation). The value of fold-increase in +1FS frequency is shown for each construct. (e) Synthetic lethality oftrmD−andefp−.S. typhimuriumstrains carryingefp+or efp−and/or a temperature-sensitive (ts) allele oftrmD17were grown at 30 or 44 °C, the permissive or the non-permissive temperature, respectively. Among total E. coli sense codons, CC[C/U]-[C/U] occur ∼ 2,300 times, the majority of which are within the first 100 codons of protein-coding genes ( Supplementary Table 1 ). Some of these sequences are directly adjacent to the start codon, whereas others are within a short distance from the start ( Supplementary Fig. 1a,b ). Notably, the CC[C/U]-[C/U] sequences are read by the GGG and UGG isoacceptors of tRNA Pro , both of which have on the 3' side of the anticodon an m 1 G37, where the N 1 of the G37 base is methylated. Although m 1 G37 is known to suppress +1FS errors [5] , the mechanism is unresolved, because the methylation does not interfere with the anticodon–codon base pairing interaction. Between the two isoacceptors of tRNA Pro , the UGG isoacceptor is of high interest, because it is essential for cell growth [6] and it is capable of reading all Pro codons, including the CC[C/U]-[C/U], through the use of an additional modification cmo 5 at the wobble base U34. The critical barrier to understanding the mechanism of producing and suppressing +1FS errors is the lack of quantitative assays to monitor errors. We thus developed quantitative assays to measure intracellular translation of lacZ containing the CCC-C sequence as an example of the slippery motif. We found that early rounds of peptide synthesis are more prone to +1FS errors than later rounds, with translation at the second codon being the most shift-prone. We then developed kinetic assays to measure the formation of +1FS errors in vitro , with a view towards elucidating the ribosome reaction steps that are shift-prone. We identified two shift-prone mechanisms: a slow mechanism during tRNA Pro stalling at the P-site next to an empty A-site and a fast mechanism during tRNA Pro translocation into the P-site. Although the slow mechanism was implicated by genetic studies [2] , [7] , [8] , [9] and is relevant in nutrient starvation, the fast mechanism is a threat to cells in the normal growth condition. We found that, among natural post-transcriptional modifications in tRNA Pro , m 1 G37 is the major determinant to suppress +1FS errors; however, although it is dominant in UGG tRNA Pro , it requires the assistance of the translation factor EF-P to suppress errors of GGG tRNA Pro . This latter finding expands the biological scope of EF-P, best known for relieving ribosomes from stalling at poly-Pro sequences [10] , [11] . The action of both m 1 G37 and EF-P is strongest when CC[C/U]-[C/U] occur at the second codon, emphasizing the importance of safeguarding the ribosome for the first round of protein synthesis before it moves downstream. Together, this work highlights the prevalent and dynamic nature of tRNA shifting and the importance of m 1 G37 and EF-P to suppress shifts. The second codon is prone to +1FS errors in vivo To determine whether the placement of CCC-C relative to the start codon affects the propensity of +1FS errors inside E. coli cells, we created several constructs of the reporter lacZ , each with only one CCC-C in the entire reading frame. In the ORF2 construct, the CCC-C was inserted to the second codon, whereas in the ORF5, ORF10, ORF20, ORF60 and ORF124 constructs, it was inserted to codon 5, 10, 20, 60 and 124, respectively ( Fig. 1a ). In each construct, the CCC triplet was followed by a moderately abundant codon; for example, the CCC at position 124 was followed by the codon CAC naturally present in lacZ . With each insertion, restoration of the reading frame and synthesis of an active β-galactosidase (β-gal) required a +1FS event at the insertion site. We defined the frequency of the +1FS event by measuring the β-gal activity produced from cells expressing the CCC-C construct relative to cells expressing an in-frame insertion of CCC. To test how the +1FS event is influenced by codon context, we created two additional constructs ORF124CGG and ORF124UGG, where the CCC at position 124 was followed in the 0-frame by rare codons CGG and UGG, respectively. Figure 1: Suppression of cellular +1FS errors by m 1 G37 and EF-P. ( a ) Suppression of +1FS errors was monitored using lacZ reporter genes containing the CCC-C frameshift site (in red) adjacent to the AUG start codon or further downstream. Examples are shown for the Open Reading Frame (ORF) 2 construct with the CCC-C at the 2nd codon position and the ORF124 construct with the CCC-C at the 124th codon position. Normal translation at each CCC-C site would result in premature termination of β-gal synthesis (indicated by the symbol *) unless a +1FS event occurred with tRNA Pro . The +1FS frequency is expressed as the ratio of β-gal of the +1-frame reporter with the CCC-C sequence over the in-frame reporter with the CCC sequence. ( b ) Measurement of +1FS frequency of each reporter in an E. coli trmD-KO strain with and without the synthesis of m 1 G37. This trmD-KO strain was maintained viable by expressing the human counterpart trm5 on an arabinose-controlled expression plasmid. The m 1 G37+ condition was achieved with 0.2% (w/v) arabinose, whereas the m 1 G37- condition was achieved without arabinose. ( c ) Measurement of +1FS frequency of each reporter construct in an isogenic pair of E. coli efp + versus efp − strains. ( d ) Measurement of +1FS frequency of ORF2 and ORF10 in the E. coli efp − strain complemented by WT or K34A mutant of EF-P co-expressed with yjeA and yjeK . In b – d , each +1FS frequency is the average of at least three independent measurements, with the errors showing s.d. (standard deviation). The value of fold-increase in +1FS frequency is shown for each construct. ( e ) Synthetic lethality of trmD − and efp − . S. typhimurium strains carrying efp + or efp − and/or a temperature-sensitive ( ts ) allele of trmD [17] were grown at 30 or 44 °C, the permissive or the non-permissive temperature, respectively. Full size image To evaluate the role of m 1 G37 in suppressing the +1FS event, we created an E. coli trmD-KO (knockout) strain, where the trmD gene for the enzymatic synthesis of m 1 G37 was disrupted, and because of the growth-essentiality of the gene [12] we maintained cell viability by expressing the human counterpart trm5 gene [13] from an arabinose promoter. Upon removal of arabinose, the trmD-KO strain lost the ability to synthesize m 1 G37, although the pre-existing m 1 G37 kept cells alive for 5–6 h. During this time window, the +1FS frequency was measured in cells without synthesis of m 1 G37 relative to cells with synthesis. Translation of the CCC-C involved both GGG and UGG tRNA Pro , so the +1FS frequency reflected the effect of both. Unexpectedly, even when m 1 G37 synthesis was active, the +1FS frequency was already twofold higher at the second codon relative to later codons in constructs where the CCC-C was followed by a moderately abundant codon ( Fig. 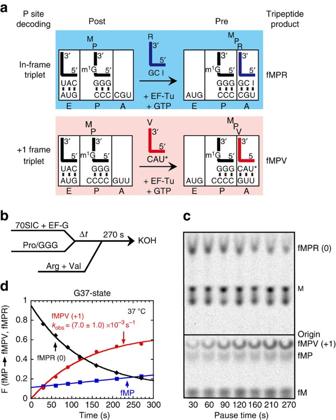Figure 2: Assays for +1FS errors of GGG tRNAProat the second codon. (a) Diagram of two possible pairing states of fMP-tRNAPro/GGGat the P-site of a stalled post-translocation complex and the corresponding pre-translocation complexes after one round of peptide bond formation on anE. coli70SIC programmed with the mRNA AUG-CCC-CGU-U. Each tRNA is shown in the L shape with the anticodon specified. The letter I in the anticodon of tRNAArgdenotes inosine and the letter U* in the anticodon of tRNAValdenotes cmo5U; both are capable of pairing with U. While in-frame triplet pairing of tRNAProin the P-site would direct formation of fMPR, +1-frame pairing would direct formation of fMPV. Occupancy of the E site by the deacylated tRNAfMetis probably short-lived. (b) An fMP-post-translocation complex was formed via rapid mixing of a 70SIC with the ternary complex of G37-state tRNAPro/GGGin the presence of EF-G. Over a time course to allow tRNAPro/GGGto shift into the +1-frame, aliquots were mixed with ternary complexes of tRNAArg(Arg) and tRNAVal(Val) to support tripeptide synthesis, followed by quenching with KOH. (c) Electrophoretic TLC of quenched reactions, showing conversion of fMP to fMPR (the 0-frame product) and fMPV (the +1-frame product). Remaining substrates fM and M are indicated. (d) Plots of the fractional conversion of fMP to fMPR and to fMPV over time. The F in theyaxis is the fractional synthesis of fMPR or fMPV from total fMP molecules, including reactive and non-reactive fMP molecules. Please note that data here were collected at 37 °C, whereas data in the rest of the experiments in this work were collected at room temperature (20 °C). At equilibrium at 37 °C, the percentage of the G37-state tRNAProin the +1-frame was 67%, whereas at 20 °C it was 26% (Fig. 4b). This effect indicates that tRNA slippage is favored by higher temperature. Error range of curve fitting is denoted for fMPV formation. 1b and Supplementary Table 2a ). When m 1 G37 synthesis was inactivated, the +1FS frequency increased dramatically by eightfold for ORF2 but only by two- to fourfold for other constructs, indicating a specific role of m 1 G37 in suppressing +1FS errors at the second codon. For constructs where the CCC-C was followed by a rare codon, the basal level of +1FS errors was higher relative to an abundant codon and error suppression by m 1 G37 was dependent on the nature of the codon: inactivation of m 1 G37 synthesis increased errors by 1.5-fold for ORF124CGG but by 4-fold for ORF124UGG. Thus, regardless of where the CCC-C appears relative to the start codon, m 1 G37 is important for suppressing +1FS errors, although its strongest effect was at the second codon. Translation of the second codon requires stable positioning of the initiator fMet-tRNA fMet , which in bacteria is enforced by EF-P, the translation factor that stimulates the first peptide bond formation [10] . Because elimination of EF-P in bacteria does not cause cell death, we compared an E. coli efp − strain with the isogenic efp + strain to determine its role in reading-frame maintenance ( Fig. 1c and Supplementary Table 2b ). In efp + cells, the +1FS frequency in our lacZ assay was the highest when the CCC-C was placed at the second codon, but it gradually decreased as the CCC-C moved downstream. In efp − cells, the +1FS frequency increased most dramatically at the second codon, but only moderately at later codons. When the +1FS frequency was elevated due to the placement of CCC before a rare codon, the removal of EF-P further increased errors at both ORF124CGG and ORF124UGG. Notably, E. coli EF-P contains a K34 that is hydroxylated and β-lysylated [14] , [15] , [16] . This modified K34 was important for the shift-suppression activity; the +1FS frequency rose by 3.8-fold at the second codon and by 4.6-fold at the tenth codon in cells expressing the K34A mutant of EF-P ( Fig. 1d and Supplementary Table 2c ). Collectively, these data revealed a previously unrecognized role of EF-P in suppressing +1FS errors, showing that it has the strongest error-suppression effect at the second codon. In m 1 G37 + or EF-P + cells, the +1FS frequency of 0.4–1.0% when the CCC-C was placed at the second codon was high relative to the average frequency of 0.003% in bacteria [1] . This points to the propensity of the ribosome to +1-frameshifting at the second codon and it may explain why E. coli has only four genes with CCC-C at the second codon, including one growth-essential gene lolB (for localization of lipoproteins to outer-membrane) and three non-essential genes pncA (nicotinamide deamidase, Supplementary Fig. 1b ), ygcP (for anti-terminator regulation) and ptrA (for a zinc metalloprotease). Our result suggests that translation of each of these genes requires both m 1 G37 and EF-P to minimize +1FS errors. This is supported by analysis of the protein product of pncA , showing that the enzyme activity in cell lysates was reduced by 2.5-fold upon elimination of m 1 G37 and by 2.3-fold upon elimination of EF-P. A similar reduction upon inactivation of m 1 G37 synthesis was also observed in a trmD TS (temperature sensitive) [17] strain ( Supplementary Fig. 1c ). The importance of both m 1 G37 and EF-P for reading frame maintenance is further emphasized by the synthetic lethality of a double mutant harbouring the trmD TS and efp − alleles ( Fig. 1e ). The high +1FS frequency upon inactivation of m 1 G37 (at 8.3%) may thus indicate a threshold for cell survival. Kinetic analysis of +1FS errors To determine the kinetics of +1-frameshifting and its speed relative to peptide bond formation, we developed assays for monitoring shift errors using purified ribosomal components. Both GGG and UGG tRNA Pro were examined in three states: (i) the G37-state transcript, lacking any post-transcriptional modifications, (ii) the m 1 G37-state transcript, containing only the TrmD-introduced modification and (iii) the native-state isolated from cells containing all natural modifications ( Supplementary Fig. 2 ). Stoichiometric levels of m 1 G37 in the m 1 G37- and native-state of both tRNAs were confirmed by RNase T1 analysis ( Supplementary Fig. 3a ). Two additional states of UGG tRNA Pro were also examined: (iv) the G37-state and (v) the ho 5 U34-state (the precursor of the cmo 5 U34 state) [18] in an otherwise native tRNA. These two states were isolated from E. coli cells deficient in the synthesis of m 1 G37 and in the conversion of ho 5 U34 to cmo 5 U34, respectively. To study the high propensity of +1FS errors at the second codon, we programmed an E. coli 70SIC with an mRNA starting with the sequence AUG- CCC - C GU-U, where the CCC-C was placed at the second codon. Using GGG tRNA Pro as an example, the post-translocation complex after one round of peptide bond formation contained deacylated tRNA fMet in the E-site, fMet-Pro (fMP)-tRNA Pro in the P-site and an empty A-site ( Fig. 2a ). Pairing of tRNA Pro/GGG in the 0-frame would position the Arg CGU codon in the A-site, whereas pairing in the +1-frame would position the Val GUU codon in the A-site. By incubating the stalled complex over time to allow tRNA Pro/GGG to shift into the +1-frame, we determined the state of shifting by simultaneously adding ternary complexes (TCs) of tRNA Arg and tRNA Val to allow for a second round of peptide bond formation ( Fig. 2b ). The 0-frame pairing of tRNA Pro/GGG would generate fMet-Pro-Arg (fMPR), whereas the +1-frame pairing would generate fMet-Pro-Val (fMPV). Analysis of the two products by electrophoretic thin-layer chromatography (TLC; Fig. 2c ) showed a slow but steady increase of the +1-frame product fMPV and a concomitant reduction of the 0-frame product fMPR ( Fig. 2d ). This result, together with toeprint analysis ( Supplementary Fig. 3b ), supports a time-dependent shift of tRNA Pro/GGG into the +1-frame. Although the rate of synthesis of the +1-frame product fMPV was slow (10 −2 –10 −3 s −1 ), it was still ∼ 100-fold faster relative to mis-incorporation of Val due to tRNA Val mis-pairing at the Arg CGU codon or out-of-frame pairing at the Val GUU codon [19] ( Supplementary Fig. 4 ). Thus, the synthesis of fMPV from fMP was attributed to the peptide bond formation after tRNA Pro/GGG shifted into the +1-frame, rather than the mis-coding by tRNA Val . Figure 2: Assays for +1FS errors of GGG tRNA Pro at the second codon. ( a ) Diagram of two possible pairing states of fMP-tRNA Pro/GGG at the P-site of a stalled post-translocation complex and the corresponding pre-translocation complexes after one round of peptide bond formation on an E. coli 70SIC programmed with the mRNA AUG-CCC-CGU-U. Each tRNA is shown in the L shape with the anticodon specified. The letter I in the anticodon of tRNA Arg denotes inosine and the letter U* in the anticodon of tRNA Val denotes cmo 5 U; both are capable of pairing with U. While in-frame triplet pairing of tRNA Pro in the P-site would direct formation of fMPR, +1-frame pairing would direct formation of fMPV. Occupancy of the E site by the deacylated tRNA fMet is probably short-lived. ( b ) An fMP-post-translocation complex was formed via rapid mixing of a 70SIC with the ternary complex of G37-state tRNA Pro/GGG in the presence of EF-G. Over a time course to allow tRNA Pro/GGG to shift into the +1-frame, aliquots were mixed with ternary complexes of tRNA Arg (Arg) and tRNA Val (Val) to support tripeptide synthesis, followed by quenching with KOH. ( c ) Electrophoretic TLC of quenched reactions, showing conversion of fMP to fMPR (the 0-frame product) and fMPV (the +1-frame product). Remaining substrates fM and M are indicated. ( d ) Plots of the fractional conversion of fMP to fMPR and to fMPV over time. The F in the y axis is the fractional synthesis of fMPR or fMPV from total fMP molecules, including reactive and non-reactive fMP molecules. Please note that data here were collected at 37 °C, whereas data in the rest of the experiments in this work were collected at room temperature (20 °C). At equilibrium at 37 °C, the percentage of the G37-state tRNA Pro in the +1-frame was 67%, whereas at 20 °C it was 26% ( Fig. 4b ). This effect indicates that tRNA slippage is favored by higher temperature. Error range of curve fitting is denoted for fMPV formation. Full size image Additional data validated the biological relevance of these kinetic assays. First, a C31A mutation in the G37-state tRNA Pro/GGG elevated the amplitude of the shift to 50% ( Supplementary Fig. 5 ), consistent with a genetic study [20] showing that disrupting the 31–39 base pair of tRNA Pro increased +1FS errors. Second, the +1-shift of tRNA Pro/GGG in a stalled post-complex also occurred with other mRNAs, such as the AUG-CCC-CUU sequence ( Supplementary Fig. 6 ). Third, these assays revealed specific shifting features of each tRNA Pro . For GGG tRNA Pro , the base identity following the CCC triplet was a strong determinant of the shift, whereas for UGG tRNA Pro , its propensity of shifting was independent of the base identity following the CCC triplet ( Supplementary Fig. 7 ). Ribosome active for catalyzing peptidyl transfer on +1-frame We found that with the G37-state tRNA Pro/GGG , despite its shift to the +1-frame, the ribosome was fully active for the next peptide bond formation. Specifically, after the shift reached equilibrium, addition of TCs of both tRNA Arg and tRNA Val showed faster synthesis of the +1-frame fMPV product relative to the 0-frame fMPR product ( Fig. 3a,b ), indicating that peptidyl transfer was not perturbed by the shift. In addition, the peptide on the shifted tRNA was not removed by the ribosome or release factors ( Supplementary Fig. 8 ), indicating that +1FS errors were not subject to the ribosome post-peptidyl-transfer quality control that removes mis-incorporation errors [21] . The faster synthesis of fMPV may reflect a more favourable event for peptidyl transfer to Val [22] and/or for the base-pairing context of the codon–anticodon interaction. Importantly, the faster synthesis of fMPV was also observed with the m 1 G37- or the native-state of the tRNA ( Fig. 3b ), indicating that it was independent of the state of tRNA modification. Instead, the amplitude of the shift decreased from 23% with the G37-state to 11% and 9% with the m 1 G37- and native-state, respectively. Because the m 1 G37- and the native-state exhibited virtually identical error reduction, the single m 1 G37 modification is the major determinant and its action alone is as effective as the sum of all modifications. 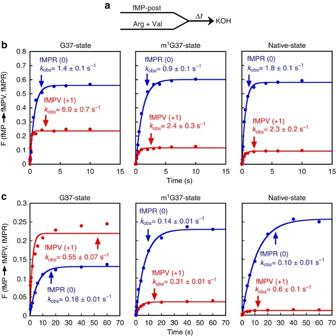Figure 3: Peptide bond formation by a post-translocation complex with GGG or UGG tRNAProstalled at the P-site. (a) Kinetic scheme for measurement ofkobsof peptide bond formation upon rapid mixing of excess ternary complexes of tRNAArgand tRNAVal(molar ratio of 1:1) with a stalled post-initiation complex carrying fMP-tRNAPro/GGGor fMP-tRNAPro/UGGin the P-site. The coding mRNA sequence was AUG-CCC-CGU-U. (b) Measurement of the fractional conversion F of total fMP molecules to the in-frame fMPR product (blue) and to the +1-frame fMPV product (red) over time for G37- (left), m1G37- (middle) and native-state (right) tRNAPro/GGG, showing the rate constant of conversion (kobs) for each. Yields of the respective tripeptides did not change when the molar ratio of tRNAArgto tRNAValwas varied from 1:5 to 5:1 or when each incoming tRNA ternary complex was added separately to a limiting amount of the post-translocation complex. (c) Similar analysis conducted with tRNAPro/UGG(anticodon presented 5' to 3') in the P-site of the post-translocation complex. Error range of the curve fitting is denoted. Figure 3: Peptide bond formation by a post-translocation complex with GGG or UGG tRNA Pro stalled at the P-site. ( a ) Kinetic scheme for measurement of k obs of peptide bond formation upon rapid mixing of excess ternary complexes of tRNA Arg and tRNA Val (molar ratio of 1:1) with a stalled post-initiation complex carrying fMP-tRNA Pro/GGG or fMP-tRNA Pro/UGG in the P-site. The coding mRNA sequence was AUG-CCC-CGU-U. ( b ) Measurement of the fractional conversion F of total fMP molecules to the in-frame fMPR product (blue) and to the +1-frame fMPV product (red) over time for G37- (left), m 1 G37- (middle) and native-state (right) tRNA Pro/GGG , showing the rate constant of conversion ( k obs ) for each. Yields of the respective tripeptides did not change when the molar ratio of tRNA Arg to tRNA Val was varied from 1:5 to 5:1 or when each incoming tRNA ternary complex was added separately to a limiting amount of the post-translocation complex. ( c ) Similar analysis conducted with tRNA Pro/UGG (anticodon presented 5' to 3') in the P-site of the post-translocation complex. Error range of the curve fitting is denoted. Full size image The effect of m 1 G37 in the UGG isoacceptor tRNA Pro (tRNA Pro/UGG ) is most remarkable. Although the ribosome was active with all three states of the tRNA for synthesis of fMPV, the fractional synthesis decreased markedly from 22% with the G37-state to 4% with the m 1 G37- and to 2% with the native-state ( Fig. 3c ), each accompanied by more than a 100-fold reduction in kinetics of +1 frameshifting (see Fig. 5b ). Thus, the single m 1 G37 is the major determinant to suppress +1FS errors, suggesting that all other modifications in the native-state, including the cmo 5 U34, have little effect. Indeed, substitution of cmo 5 U34 with ho 5 U34 in an otherwise native-state had no effect on the amplitude of the shift, whereas substitution of m 1 G37 with G37 in the native-state greatly increased the amplitude ( Supplementary Fig. 9 ). Error suppression at the second codon Because the second codon is most shift-prone, we determined the action of m 1 G37 and EF-P at this position. To determine the m 1 G37 effect, we compared the kinetics of tRNA Pro shifting into the +1-frame in the G37-state and in the m 1 G37-containing native-state. In a ribosome complex on the mRNA AUG-CCC-C sequence with GGG tRNA Pro stalled in the P-site, we showed that the tRNA shifting into the +1-frame was slow ( k obs =10 −3 –10 −2 s −1 , Fig. 4a,b ) relative to peptide bond formation ( ∼ 1 s −1 ; Supplementary Fig. 10 ), indicating that such shifts are rare during active protein synthesis but are induced when the A-site is empty. A slow shift was also observed with the native-state, indicating that m 1 G37 does not suppress the kinetics of shift of this tRNA. In fact, the k obs of shift of the native-state GGG tRNA Pro was generally faster relative to the G37-state, indicating that the full complement of natural modifications in the native-state rendered the tRNA kinetically more competent on the ribosome. Importantly, although m 1 G37 did not reduce the kinetics of shift, it reduced the amplitude, from 26% with the G37-state to 8.1% with the native state. 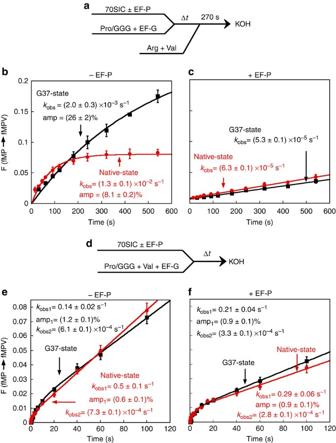Figure 4: Formation of +1FS errors by GGG tRNAProat the second codon. (a) The kinetic scheme to measure the rate of +1FS formation by fMP-tRNAPro/GGGstalled at the P-site of a post-translocation complex on the template AUG-CCC-CGU-U. A 70SIC was mixed with Pro-tRNAPro/GGGand EF-G to form a stalled post-translocation complex, which was sampled over time by mixing with excess ternary complexes of tRNAArgand tRNAVal(molar ratio of 1:1). After 270 s of peptide synthesis, each secondary reaction was quenched and the peptides analysed. (b) Time course of the fractional conversion F from total fMP molecules to fMPV molecules, showing the kinetics of +1-frameshifting by the G37- (black) and native-state (red) of tRNAPro/GGGat 20 °C. (c) Analysis as inbbut in the presence of EF-P (10 μM). (d) The kinetic scheme to measure the rate of +1FS formation by fMP-tRNAPro/GGGwhen a 70SIC was rapidly mixed with ternary complexes of tRNAProand tRNAValin the presence of EF-G. (e) Biphasic kinetics were observed for +1FS by both the G37- (black) and native-state (red) tRNAPro/GGG. (f) Analysis as inebut in the presence of EF-P (10 μM). Thekobsand amplitude of each shift are indicated, each as the average of at least three independent measurements. Error bars denote s.d. Figure 4: Formation of +1FS errors by GGG tRNA Pro at the second codon. ( a ) The kinetic scheme to measure the rate of +1FS formation by fMP-tRNA Pro/GGG stalled at the P-site of a post-translocation complex on the template AUG-CCC-CGU-U. A 70SIC was mixed with Pro-tRNA Pro/GGG and EF-G to form a stalled post-translocation complex, which was sampled over time by mixing with excess ternary complexes of tRNA Arg and tRNA Val (molar ratio of 1:1). After 270 s of peptide synthesis, each secondary reaction was quenched and the peptides analysed. ( b ) Time course of the fractional conversion F from total fMP molecules to fMPV molecules, showing the kinetics of +1-frameshifting by the G37- (black) and native-state (red) of tRNA Pro/GGG at 20 °C. ( c ) Analysis as in b but in the presence of EF-P (10 μM). ( d ) The kinetic scheme to measure the rate of +1FS formation by fMP-tRNA Pro/GGG when a 70SIC was rapidly mixed with ternary complexes of tRNA Pro and tRNA Val in the presence of EF-G. ( e ) Biphasic kinetics were observed for +1FS by both the G37- (black) and native-state (red) tRNA Pro/GGG . ( f ) Analysis as in e but in the presence of EF-P (10 μM). The k obs and amplitude of each shift are indicated, each as the average of at least three independent measurements. Error bars denote s.d. Full size image The amplitude at 26% of the G37-state GGG tRNA Pro is notable, indicating that one-quarter of the post complexes at the second codon CCC-C occupy the +1-frame at equilibrium. Even with the amplitude reduced to 8.1% by m 1 G37, the level is still high (almost the level that challenges cell survival). We showed that the addition of EF-P effectively suppressed the amplitude to the background and reduced the kinetics by more than a 100-fold from 10 −2 –10 −3 to 10 −5 s −1 ( Fig. 4c ). This error suppression by EF-P was dependent on the β-lysyl K34; an EF-P produced from cells co-expressing the β-lysylation activity [23] was effective in suppressing the shift, whereas the K34A mutant ( Supplementary Fig. 11 ) and the protein without the β-lysyl modification of K34 were less effective. Notably, β-lysyl EF-P reduced the kinetics of shift by 40-fold for the G37-state and by 200-fold for the native-state ( Fig. 4b,c ), showing a stronger effect on the m 1 G37-containing native-state. We sought to determine whether there existed other translational steps that would permit a faster shift relative to the shift from the P-site. In a concerted assay that monitored successive activities of GGG tRNA Pro from decoding at the A-site to translocation into the P-site, we observed biphasic shift kinetics ( Fig. 4d,e ). Both the G37- and native-state displayed similar kinetics, with a fast k obs1 followed by a slow k obs2 . Because the slow k obs2 (10 −3 –10 −4 s −1 ) was comparable to the rate of tRNA shifting from the P-site, we attributed the fast k obs1 (0.1–0.2 s −1 ) to the tRNA shifting before arrival at the P-site. This assignment was supported by the observation that occupancy of the 0-frame tRNA Arg at the A-site suppressed the slow shift but not the fast shift ( Supplementary Fig. 12 ). Given the lack of shifting in the A-site [24] , [25] and the lack of robust peptide bond formation when decoding an out-of-frame triplet ( Supplementary Fig. 4 ), we suggest that the fast k obs1 reports on the tRNA shifting during translocation into the P-site. Both m 1 G37 and EF-P had small effects in reducing the amplitude of the fast shift ( Fig. 4e,f ). This shift is of interest, because its k obs1 is comparable to the rate of peptide bond formation and thus it can affect reading frame accuracy during active protein synthesis. Also, its association with tRNA translocation has parallel to that found in programmed −1 frameshifting [26] , [27] . UGG tRNA Pro differs from its GGG counterpart in both the slow and fast shift. The slow shift of UGG tRNA reached a higher level, but m 1 G37 alone reduced it to background and decreased the kinetics from 10 −3 to 10 −5 s −1 ( Fig. 5a,b ). This dual role of m 1 G37 in UGG tRNA is in contrast to its single role in reducing the amplitude in GGG tRNA. EF-P had little effect on the slow shift of UGG tRNA in all three states ( Fig. 5c ), in contrast to its strong effects on GGG tRNA. Conversely, the fast shift of UGG tRNA also reached a higher level relative to GGG tRNA ( Fig. 5d,e ), indicating that UGG tRNA can have a stronger impact during active protein synthesis. Both m 1 G37 and EF-P had small effects on the amplitude of the fast shift ( Fig. 5c,f ). 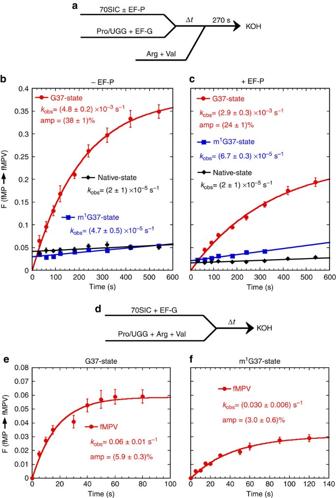Figure 5: Formation of +1FS errors by UGG tRNAProat the second codon. (a) Kinetic scheme to measure the rate of +1FS formation by fMP-tRNAPro/UGGstalled at the P-site of a post-translocation complex on the template AUG-CCC-CGU-U. Sampling was the same as inFig. 4a. (b) Time course of the fractional conversion F from total fMP molecules to fMPV molecules, showing the kinetics of +1FS by the G37- (red), m1G37- (blue) and native-state (black) of tRNAPro/UGG. (c) Analysis as inbbut in the presence of EF-P (10 μM). (d) Kinetic scheme to measure the rate of +1FS formation by fMP-tRNAPro/UGGwhen a 70SIC was rapidly mixed with ternary complexes of tRNAProand tRNAValin the presence of EF-G. (e) Kinetics of +1FS formation by the G37-state tRNAPro/UGG. (f) Kinetics of +1FS formation by the m1G37-state tRNAPro/UGG. Thekobsand amplitude of each shift are indicated, each as the average of at least three independent measurements. Error bars denote s.d. Figure 5: Formation of +1FS errors by UGG tRNA Pro at the second codon. ( a ) Kinetic scheme to measure the rate of +1FS formation by fMP-tRNA Pro/UGG stalled at the P-site of a post-translocation complex on the template AUG-CCC-CGU-U. Sampling was the same as in Fig. 4a . ( b ) Time course of the fractional conversion F from total fMP molecules to fMPV molecules, showing the kinetics of +1FS by the G37- (red), m 1 G37- (blue) and native-state (black) of tRNA Pro/UGG . ( c ) Analysis as in b but in the presence of EF-P (10 μM). ( d ) Kinetic scheme to measure the rate of +1FS formation by fMP-tRNA Pro/UGG when a 70SIC was rapidly mixed with ternary complexes of tRNA Pro and tRNA Val in the presence of EF-G. ( e ) Kinetics of +1FS formation by the G37-state tRNA Pro/UGG . ( f ) Kinetics of +1FS formation by the m 1 G37-state tRNA Pro/UGG . The k obs and amplitude of each shift are indicated, each as the average of at least three independent measurements. Error bars denote s.d. Full size image Error suppression at the third codon We evaluated the effect of m 1 G37 and EF-P at the third codon as a representative of later codons. In a stalled ribosome complex on an mRNA starting with AUG-UAU- CCC - C GU-U, the G37-state of GGG tRNA Pro exhibited a slow shift into the +1-frame ( Fig. 6a,b ), although with a k obs faster and an amplitude higher relative to its placement at the second codon. Although m 1 G37 had no effect on the kinetics or amplitude of the shift, β-lysyl EF-P had a small effect on both, reducing the kinetics from 1.9 × 10 −2 to 7.0 × 10 −3 s −1 and the amplitude from 43 to 34% ( Fig. 6c ). These are smaller effects relative to those at the second codon. In the concerted assay with both tRNA Arg and tRNA Val present, we observed no evidence of fast shift. When the same reaction was conducted with only tRNA Val present, we observed single-phase kinetics with k obs of the shift similar to that of the slow shift ( Fig. 6d–f ). Here, m 1 G37 had no effect on the kinetics, whereas EF-P had a small effect on both the kinetics and amplitude, consistent with the nature of slow shift from the P-site. 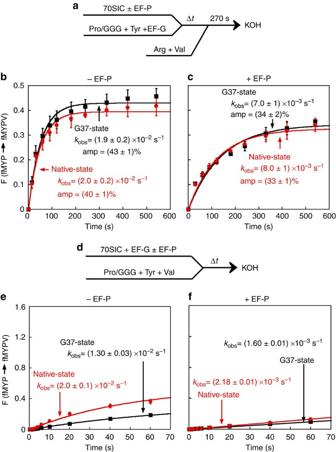Figure 6: Formation of +1FS errors by GGG tRNAProat the third codon. (a) Kinetic scheme to measure the rate of +1FS formation by fMYP-tRNAPro/GGGstalled at the P-site of a post-translocation complex on the template AUG-UAU-CCC-CGU-U. A 70SIC was mixed with ternary complexes of tRNATyrand tRNAPro/GGGin the presence of EF-G to form a stalled post complex, which was sampled over time by mixing with excess ternary complexes of tRNAArgand tRNAVal(molar ratio of 1:1). After 270 s of peptide synthesis, each reaction was quenched and the peptides were analysed. (b) Time course of the fractional conversion F from total fMYP molecules to fMYPV molecules, showing the kinetics of +1FS by the G37- (black) and native-state (red) of tRNAPro/GGG. (c) Analysis as inbbut in the presence of EF-P (10 μM). (d) The kinetic scheme to measure the rate of +1FS formation by fMYP-tRNAPro/GGGwhen a 70SIC was rapidly mixed with ternary complexes of tRNATyr, tRNAPro/GGGand tRNAValin the presence of EF-G. (e) Kinetics of +1FS formation by G37- (black) and native-state (red) tRNAPro/GGGwere determined. (f) Analysis as inebut in the presence of EF-P (10 μM). Thekobsand amplitude of each shift are indicated, each as the average of at least three independent measurements. Error bars denote s.d. Figure 6: Formation of +1FS errors by GGG tRNA Pro at the third codon. ( a ) Kinetic scheme to measure the rate of +1FS formation by fMYP-tRNA Pro/GGG stalled at the P-site of a post-translocation complex on the template AUG-UAU-CCC-CGU-U. A 70SIC was mixed with ternary complexes of tRNA Tyr and tRNA Pro/GGG in the presence of EF-G to form a stalled post complex, which was sampled over time by mixing with excess ternary complexes of tRNA Arg and tRNA Val (molar ratio of 1:1). After 270 s of peptide synthesis, each reaction was quenched and the peptides were analysed. ( b ) Time course of the fractional conversion F from total fMYP molecules to fMYPV molecules, showing the kinetics of +1FS by the G37- (black) and native-state (red) of tRNA Pro/GGG . ( c ) Analysis as in b but in the presence of EF-P (10 μM). ( d ) The kinetic scheme to measure the rate of +1FS formation by fMYP-tRNA Pro/GGG when a 70SIC was rapidly mixed with ternary complexes of tRNA Tyr , tRNA Pro/GGG and tRNA Val in the presence of EF-G. ( e ) Kinetics of +1FS formation by G37- (black) and native-state (red) tRNA Pro/GGG were determined. ( f ) Analysis as in e but in the presence of EF-P (10 μM). The k obs and amplitude of each shift are indicated, each as the average of at least three independent measurements. Error bars denote s.d. Full size image In contrast, the G37-state of UGG tRNA Pro is subject to both slow and fast shifts at the third codon ( Supplementary Fig. 13 ). In the slow shift, m 1 G37 reduced the amplitude of the shift by a small effect, but EF-P had no effect, whereas in the fast shift, neither had an effect. Importantly, the detection of fast shifts with UGG tRNA is in contrast to the absence of fast shifts of GGG tRNA. This indicates that UGG tRNA is responsible for fast shifts at the third and later codons, consistent with its major role in driving shifts in genetic analysis [20] . Cell viability depends on a balance between rapid protein synthesis and accurate reading-frame maintenance. Here we provide insight into this balance by elucidating the molecular mechanisms governing +1-frameshifting of GGG and UGG tRNA Pro at the CCC-C sequence ( Supplementary Table 3 ). We have identified two mechanisms: the fast shift during tRNA translocation into the P-site and the slow shift during tRNA stalling next to an empty A-site ( Fig. 7 ). With the exception of the first round of elongation, the fast shift mechanism is restricted to UGG tRNA. In contrast, the slow shift mechanism is accessible to either tRNA at any round of elongation. EF-P and m 1 G37 are selective inhibitors of +1-frameshifting. Although neither factor has a strong effect on the fast shift mechanism, both exert a strong but differential effect on suppressing the slow shift. EF-P inhibits slow shifts of GGG tRNA, whereas m 1 G37 inhibits slow shifts of UGG tRNA. These data form the basis for an important conceptual advance for understanding how +1FS errors are formed and suppressed in cells. In the absence of stress, cells expressing both m 1 G37 and EF-P have low levels of +1-frameshifting at a CCC-C sequence, primarily due to fast shifts of UGG tRNA during translocation. The one exception is at the second codon, where both UGG and GGG tRNAs can slip, thus accounting for the noticeably high levels of endogenous frameshifting at this codon in our lacZ assays. However, in times of nutrient starvation, the slow shift becomes more relevant and cells lacking m 1 G37 or EF-P show elevated +1FS errors in each round of protein synthesis. 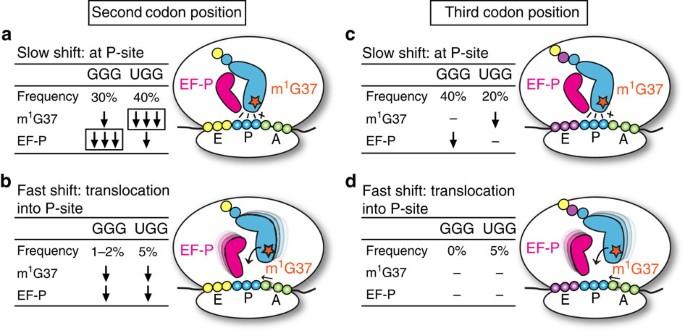Figure 7: A model of +1FS on CCC-C by GGG and UGG tRNAPro. Frequencies of +1FS on CCC-C are shown for GGG or UGG tRNAProbased on kinetic data for the G37-state of each. (a) In the post-translocation complex where CCC-C is placed at the second codon position, the high frequencies of slow shifts, due to tRNAProshifting from a stalled P-site, are suppressed primarily by m1G37 for the UGG tRNA and by EF-P for the GGG tRNA. (b) The low frequencies of fast shifts at the second codon, due to tRNAProshiftingen routeto the P-site, are suppressed by both m1G37 and EF-P for each tRNA. (c) When CCC-C is placed at the third codon position, the high frequencies of slow shifts are suppressed by m1G37 for the UGG tRNA and by EF-P for the GGG tRNA. (d) The low frequencies of fast shifts in the early elongation phase are not effectively suppressed by m1G37 or EF-P. Open arrows indicate suppression of error frequencies, whereas boxed arrows indicate suppression of both frequencies and kinetics of error formation. One arrow indicates a reduction of 2- to 3-fold, two arrows indicate 3- to 30-fold, three arrows indicate greater than 30-fold and a ‘−’ indicates less than 2-fold effects. Percent frequencies are rounded up to the closest approximation. Figure 7: A model of +1FS on CCC-C by GGG and UGG tRNA Pro . Frequencies of +1FS on CCC-C are shown for GGG or UGG tRNA Pro based on kinetic data for the G37-state of each. ( a ) In the post-translocation complex where CCC-C is placed at the second codon position, the high frequencies of slow shifts, due to tRNA Pro shifting from a stalled P-site, are suppressed primarily by m 1 G37 for the UGG tRNA and by EF-P for the GGG tRNA. ( b ) The low frequencies of fast shifts at the second codon, due to tRNA Pro shifting en route to the P-site, are suppressed by both m 1 G37 and EF-P for each tRNA. ( c ) When CCC-C is placed at the third codon position, the high frequencies of slow shifts are suppressed by m 1 G37 for the UGG tRNA and by EF-P for the GGG tRNA. ( d ) The low frequencies of fast shifts in the early elongation phase are not effectively suppressed by m 1 G37 or EF-P. Open arrows indicate suppression of error frequencies, whereas boxed arrows indicate suppression of both frequencies and kinetics of error formation. One arrow indicates a reduction of 2- to 3-fold, two arrows indicate 3- to 30-fold, three arrows indicate greater than 30-fold and a ‘−’ indicates less than 2-fold effects. Percent frequencies are rounded up to the closest approximation. Full size image The second codon is unique for its high susceptibility to fast shifts of both UGG and GGG tRNAs. This may be due to its association with the first translocation event, which has several unique features. One is the absence of an E-site tRNA, which can promote reading-frame errors [28] , [29] ; the second is the association of the ribosome complex with the Shine-Dalgarno (SD) sequence, which can hamper the first translocation and promote tRNA shifting [30] ; and the third is the involvement of the structurally distinct initiator tRNA fMet in moving from the P- to E-site. Owing to the lack of a normal first base pair in the acceptor stem, tRNA fMet is preferentially stabilized in the classical state, rather than the hybrid state, rendering the first translocation structurally and dynamically unfavourable [31] . In contrast, translocation in later cycles has a steady occupancy of the E-site, is dissociated from the SD sequence, and engages only elongator tRNAs with conformational flexibility that is lacking in tRNA fMet . This conformational flexibility enables each elongator tRNA to readily adopt intermediate structures in the hybrid state to maintain tight contacts with the ratcheting ribosome [32] , [33] . In addition, upon moving away from the start codon, each translating ribosome narrows down the mRNA entrance channel [34] to facilitate the interaction of two strictly conserved bases in the 16S rRNA with the mRNA bases. The action of these two bases, representing pawls of the translocation ratchet, may prevent slippage of the reading frame [33] . The second codon is also highly susceptible to slow shifts. The CCC triplet itself is a rare codon prone to inducing ribosome stalling [35] and when it is followed by another rare codon, the sequence context increases the translational +1FS frequency ( Fig. 1b,c ). Protein-coding sequences often contain clusters of rare codons within the first 25 positions [36] , [37] . This is an evolutionarily conserved feature that should sensitize slippery sequences such as CCC to slow shifts, whenever a shortage of aminoacyl-tRNAs occurs. Our data emphasize the importance of m 1 G37 and EF-P for suppressing +1FS errors. Although additional factors contributing to reading-frame maintenance are possible, the strong effect of m 1 G37 and EF-P and the growth arrest upon their concurrent removal suggests that they are the major determinants to correctly position a translating ribosome throughout protein synthesis. Intriguingly, suppression of shifts by m 1 G37 and EF-P is balanced between the GGG and UGG isoacceptors. This balance is most striking for suppression of slow shifts at the second codon ( Fig. 7a ), where m 1 G37 controls UGG tRNA, whereas EF-P controls GGG tRNA, both by acting on the frequency and the kinetics of shifts. In fact, the second codon is the only place where m 1 G37 and EF-P have a dramatic effect on the kinetics of shifts, whereas in all other instances they primarily act on the frequency of shifts. For suppressing fast shifts, the two factors act similarly with either tRNA ( Fig. 7b ). At the third codon, the two factors again divide their responsibility between the two tRNAs to suppress slow shifts ( Fig. 7c ), albeit with a weaker effect relative to the second codon, and neither factor suppresses fast shifts ( Fig. 7d ). Thus, in the overall landscape of error reduction, m 1 G37 is mainly responsible for reducing slow shifts of UGG tRNA Pro , whereas EF-P is the counterpart for GGG tRNA Pro . If the ribosome stalling time at the CCC-C is long relative to peptide bond formation, then the high levels of errors at the second codon upon elimination of m 1 G37 are primarily due to slow shifts of UGG tRNA Pro , whereas they arise from slow shifts of GGG tRNA Pro upon elimination of EF-P. The preference of m 1 G37 for UGG tRNA Pro is likely a consequence of the weak anticodon pairing to the CCC codon. Because the cmo 5 modification at U34 plays little role in suppressing shifts, this tRNA must accommodate the imperfect pairing of U34, ho 5 U34 or cmo 5 U34 with C, regardless in the 0- or +1-frame. How m 1 G37 restricts the pairing to the 0-frame is therefore intriguing. We suggest that m 1 G37 enhances the quality of the imperfect U-C pairing in the 0-frame by pre-organizing the anticodon loop and by promoting new interactions with the ribosome. A recent crystal structure of CGG tRNA Pro supports the concept of pre-organization, showing that m 1 G37 enables U32 and A38 to form a new base pair in the anticodon loop [24] . An example of promoting new interactions with the ribosome is found in the structure of the ms 2 i 6 modification of A37 (2-methyl thio-N6 isopentenyl adenosine) in tRNA Phe , which prevents P-site tRNA from shifting by strengthening the codon–anticodon interaction in all three binding sites and by making new contacts with the ribosome between the P- and E-sites [34] . Understanding how m 1 G37 prevents UGG tRNA Pro from slow shifts will require new crystal structures of the tRNA in complex with a ribosome. In contrast, GGG tRNA Pro reads the CCC-C using three stable G-C base pairs regardless of the 0- or +1-frame. In this case, m 1 G37 alone is unlikely to influence the pairing frame. Instead, the tRNA recruits EF-P, which binds to the P-site tRNA on the ribosome next to the E-site [38] , with extensive interactions that can prevent slow shifts of the P-site tRNA in a way distinct from m 1 G37. This EF-P stabilization may be particularly important for GGG tRNA, because the tRNA has a rare A32-U38 base pair in the anticodon loop known to cause ribosome mis-coding [39] and it has an unpaired U30-U40 that can destabilize the anticodon stem. In each case, the structural weakness of the tRNA may be recognized and strengthened by EF-P. Both m 1 G37 and EF-P also suppress fast shifts in a tRNA-independent manner during the first translocation ( Fig. 7b ). Because our assays for fast shifts encompass successive tRNA movements from the A- to P-site, and because there is no evidence of shifting in the A-site [24] , fast shifts most likely occur at a late stage of translocation before tRNA arrival at the P-site. Here m 1 G37 can reduce fast shifts by pre-organizing the anticodon loop, whereas EF-P can help to position tRNA correctly upon entering the P-site. Although EF-P is best known for releasing stalled ribosomes from poly-Pro sequences [10] , [11] , its suppression of tRNA shifting is likely by a different mechanism, acting at a single Pro codon. The m 1 G37 methylation is conserved in all isoacceptors of tRNA Pro and in CAG tRNA Leu and CCG tRNA Arg . The propensity of each tRNA to shift at slippery sequences is high and m 1 G37 is expected to reduce such shifts and promote protein synthesis. Similarly, EF-P is conserved in bacteria and is orthologous to the archaeal and eukaryotic initiation factor 5A (a/eIF-5A) [40] . Similar to the β-lysylation of EF-P, eIF-5A has a hypusine modification that is important for the factor to bind to the ribosome and to promote protein synthesis [41] . Based on our results here that the β-lysylation of EF-P is important for reading-frame accuracy, the hypusine modification is likely to have a similar role. This work emphasizes the importance of the post-transcriptional modification of tRNA by m 1 G37 and the post-translational modification of EF-P or eIF-5A by β-lysylation or hypusine for reading-frame maintenance. Indeed, both m 1 G37 and eIF-5A are essential to cell survival, whereas EF-P is vital for robust growth of most bacteria [17] , [41] , [42] . The engagement of these two factors after the first peptide synthesis emphasizes that starting off a ribosome on the correct reading frame is an essential aspect of translation. Reagents mRNAs were transcribed with T7 RNA polymerase and purified by denaturing gel electrophoresis. Each mRNA contained a consensus SD sequence (underlined) followed by an AUG start codon (italicized). Most studies utilized mRNA1 or mRNA2 with a CCC-C sequence (in bold face) at the second or third codon position. mRNA1: 5′-GGGA AGGAGGU AAAA AUG CCCC GUUCUAAG(CAC) 7 mRNA2: 5′-GGGA AGGAGGU AAAA AUG UAU CCCC GUUCUAAG-(CAC) 6 Tight-coupled 70S ribosomes were isolated from E. coli MRE600 cells and overexpressed His-tagged E. coli initiation and elongation factors were purified on nickel-nitrilotriacetic acid columns [43] . These reagents were aliquoted before storage at −70 °C. Recombinant His-tagged E. coli EF-P bearing a β-lysyl-K34 or the K34A mutant was expressed and purified from cells [23] co-expressing efp , yjeA and yjeK and stored at −20 °C. Kinetic measurements of +1FS Peptide bond formation was measured with a reconstituted E. coli ribosome, using purified components [44] , [45] . The +1 slippage of G37-state or native-state fMP-tRNA Pro in the P-site of a stalled post-translocation complex was monitored using a two-step reaction scheme in which 70SIC (bearing 35 S-fMet-tRNA fMet ) was mixed with the TC of Pro-tRNA Pro in the presence of EF-G. Aliquots were removed over time and supplemented with TCs of Val-tRNA Val and Arg-tRNA Arg . After a fixed period (270 s) these secondary reactions were quenched with KOH and labelled peptides were resolved on electrophoretic TLC. The +1 slippage during translocation was monitored in a Kintek chemical quench apparatus by mixing 70SIC with TCs of Pro-tRNA Pro , Val-tRNA Val and Arg-tRNA Arg . The +1 slippage attributable to both translocation and P-site stalling was monitored by chemical quench in the absence of Arg-tRNA Arg . Reagent concentrations along with a more detailed protocol are presented below. Determination of +1FS frequencies Using the first round of elongation as an example, the total frequency of +1FS was determined by incubating 70SIC (templated with mRNA1) with the TC of tRNA Pro in the presence of EF-G for 500 s followed by additional 270 s incubation with excess TCs of tRNA Arg and tRNA Val . The percent of fMP converted to fMPV reflected total +1FS. The frequency of +1FS associated with translocation was determined by incubating 70SIC with TCs of tRNA Pro , tRNA Arg and tRNA Val in the presence of EF-G. The percent of fMP converted to fMPV upon completion of the reaction reflected the frequency of +1FS due to the fast mechanism. Subtraction of this frequency from the total frequency yielded the frequency of +1FS in the P-site. Charged tRNAs All of the native tRNAs used in this study were overexpressed in E. coli and affinity purified from total tRNA using biotinylated oligonucleotide probes immobilized to streptavidin sepharose [46] . In vitro transcribed tRNA Pro was prepared using T7 RNA polymerase and was purified by electrophoresis in a 12% denaturing polyacrylamide gel. For specific experiments, tRNA Pro transcript was converted to the m 1 G37-state using TrmD in the presence of AdoMet [47] . Each tRNA was enzymatically charged with its cognate amino acid using the respective aminoacyl-tRNA synthetase and then stored in 25 mM acetate buffer (pH 5.0) at −20 °C until use. Formylation of Met-tRNA fMet was carried out during the charging reaction by including methionyl-tRNA formyl transferase and the methyl donor 10-formyltetrahydrofolate (derived from folinic acid at neutral pH) [44] . The efficiency of charging was determined by doping each reaction with a small amount of radiolabelled amino acid and determining both A 260 and radioactive counts of product tRNA after removal of free amino acid, ATP and protein by phenol extraction, gel filtration through a spin column and ethanol precipitation. This methodology indicated charging efficiencies of 40% for tRNA fMet , 52% for native tRNA Pro/GGG , 17% for transcript tRNA Pro/GGG , 60% for native tRNA Pro/UGG , 18% for transcript tRNA Pro/UGG , 67% for native tRNA Arg , 48% for native tRNA Val and 25% for native tRNA Tyr . Preparation of tRNA for kinetic measurements The G37-state was synthesized by in vitro transcription, the m 1 G37-state was synthesized by treating the tRNA transcript with E. coli TrmD in the presence of AdoMet [48] and the native-state was isolated from an E. coli overexpression strain. The UGG tRNA Pro was prepared in two additional states: the (G37) native state was prepared by isolating the native-state tRNA from the temperature-sensitive ts-trmD-S88L strain [17] grown at 44 °C for 24 h to inactivate m 1 G37 synthesis, and the (ho 5 U34) native state was prepared by isolating the native-state tRNA from an cmoB -deficient E. coli strain [18] unable to convert ho 5 U34 to cmo 5 U34 (obtained from Yale E. coli Stock Center). RNase T1 digestion Methylation of G37 in native tRNA Pro/GGG and in transcript tRNA Pro/GGG and tRNA Pro/UGG that had been treated with TrmD in the presence of AdoMet was confirmed by RNAse T1 digestion followed by polyacrylamide gel electrophoresis (PAGE) analysis ( Supplementary Fig. 3 ). Each tRNA was 3'-end labelled by Bacillus stearothermophilus CCA-adding enzyme [49] in the presence of [α- 32 P]ATP at 60 °C and digested by RNase T1 for 20 min at 50 °C in 20 mM sodium citrate (pH 5.5) and 1 mM EDTA [50] . The RNA fragments generated from cleavage were separated by denaturing 7 M urea/12% PAGE and analyzed by phosphorimaging. Toeprint of ribosomal complexes Unlabelled initiation and post-translocation complexes were formed on three 96-mer mRNAs that had been prepared by in vitro transcription. The initial coding sequences of these mRNAs were (i) AUG-CCC-CGU, (ii) AUG-CCC-AGU and (iii) AUG-CCA-CGU in an otherwise identical sequence. Before analysis, post-translocation complexes were incubated 4 min at 37 °C to promote +1FS. Reverse transcription was initiated from a 5'-end labelled DNA primer complementary to the 3'-end of each mRNA, resulting in primer extension products of approximately 60 nucleotides long. Primer extension was carried out at 37 °C for 15 min in the presence of 0.6 U μl −1 of AMV-RT, 0.6 mM each dNTP, 1.2 mM ATP, 10 mM Mg(OAc) 2 and 10 mM dithiothreitol. Reactions were extracted with phenol–chloroform–isoamyl alcohol, ethanol precipitated in the presence of glycogen carrier, and analyzed on a 40-cm-long 9% PAGE/7 M urea gel. Peptide bond formation In vitro translation reactions were monitored for peptide bond formation by mixing a 70SIC or post-translocation complex with one or more incoming TCs in a Kintek RQF-3 chemical quench flow apparatus (single incubation reactions) or on the bench (single or double incubation reactions). As appropriate, EF-G and EF-P were included in the reactions. Assays were performed in Buffer A (50 mM Tris-HCl, pH 7.5, 70 mM NH 4 Cl, 30 mM KCl, 3.5 mM MgCl 2 , 1 mM dithiothreitol, 0.5 mM spermidine) at 20 °C unless otherwise indicated. Before each reaction, TCs were freshly prepared by incubating EF-Tu with 1 mM GTP in Buffer A for 15 min at 37 °C, followed by adding one or more charged elongator tRNAs to the solution in an ice bath and incubating for an additional 15 min (molar ratio of EF-Tu to charged tRNA was 1.5 to 1.0). The 70SIC was formed by incubating E. coli 70S ribosome, IF1, IF2, IF3, mRNA and 35 S-fMet-tRNA fMet (at molar ratios of 1.5, 2.0, 2.0, 2.0, 2.0 and 1.0, respectively) in Buffer A supplemented with 1 mM GTP for 25 min at 37 °C. Post-translocation complexes were formed by incubating the 70SIC with requisite TCs and EF-G at 37 °C for 2 min. Before monitoring reaction kinetics, preformed TC, 70SIC and post-translocation complex were stored in ice. Unless otherwise specified, after addition of all components the final concentrations were 0.375 μM 70S ribosome, 0.5 μM each initiation factor 1, 2 and 3, 0.25 μM 35 S-fMet-tRNA fMet , 0.5 μM mRNA, 0.5 μM each charged elongator tRNA, 0.75 μM EF-Tu per each tRNA, 2 μM EF-G, 1 mM GTP and where indicated 10 μM EF-P. Reactions were conducted at 20 °C unless otherwise specified, and were quenched by adding concentrated KOH to 0.5 M. After a brief incubation at 37 °C, aliquots of 0.65 μl were spotted onto a cellulose-backed plastic TLC sheet and electrophoresed at 1,000 V in PYRAC buffer (62 mM pyridine, 3.48 M acetic acid, pH 2.7) until the marker dye bromophenol blue reached the water–oil interface at the anode [51] . The position of the origin was adjusted to maximize separation of the expected oligopeptide products. Spots were visualized by phosphorimaging and quantified using ImageQuant (GE Healthcare) and kinetic plots were fitted using Kaleidagraph (Synergy software). Release factor assay E. coli strains overexpressing release factors (RFs) 2 and 3 were kindly provided by Dr Takuya Ueda at the University of Tokyo. The His-tagged proteins were purified using metal affinity and DEAE-sepharose CL6B (Pharmacia) columns and incubated with GTP at 37 °C just before use. Post-translocation complexes with G37-state 35 S-fMP-tRNA Pro/GGG were prepared in Buffer C [21] . The mRNA-coding region sequence was either AUG-CCC-CGU (for fMPR) or AUG-CCC-UGA (for fMP-Stop). Post-translocation complexes were incubated at 37 °C for 10 min to facilitate +1FS and then treated with (i) 30 μM RF2 and 30 μM RF3, (ii) 30 μM RF2, (iii) 0.8 M KOH or (iv) reaction buffer C. Reactions with release factors were incubated at 37 °C for 10 min and then quenched with 5% formic acid. All other reactions were quenched with KOH. Aliquots of 1 μl were subjected to electrophoretic TLC and the radioactivity signal was analysed as described for the kinetic assays. An E. coli trmD- knockout ( trmD-KO ) strain Because trmD is essential for bacterial growth, a maintenance plasmid expressing the human counterpart trm5 was made first. For this purpose, the human counterpart trm5 gene was cloned downstream from the arabinose-controlled ParaB promoter in pKD46 and the entire arabinose operon consisting of the araC repressor, the Pc promoter and the ParaB-controlled trm5 was transferred to the pACYCDuet-1 (Novagen). E. coli BL21(DE3) cells harbouring the maintenance plasmid were subjected to λ Red recombination [52] to disrupt trmD. To do this, the kanamycin gene cassette was amplified from pKD4 by PCR using the forward primer 5′-CCACCGGATAAACGGTAAAAGACGGCGCTGTGTAGGCTGGAGCTGCTTC-3′ and the reverse primer 5′-ATCCTGGGTAAACTGATATCTCGGGGGCATGGGAATTAGCCATGGTCCATATG-3′ with extensions homologous to flanking regions of the E. coli chromosomal trmD gene. The purified PCR fragment was electroporated into competent cells expressing trm5 from the maintenance plasmid and survival colonies with trmD-KO were recovered in the absence of 0.2% (w/v) arabinose. The gene replacement was confirmed by PCR using primers flanking trmD. To cure the pKD46 plasmid from the trmD-KO strain, cells were incubated at 37 °C for one or two overnights to inactivate the ts -replication origin of the plasmid. An attempt to construct a trmD-KO strain with a maintenance plasmid expressing trmD was unsuccessful. β-Galactosidase (β-gal) assay We utilized the β-gal assay to study +1FS in vivo . First, to specifically study +1FS at the position of interest, we changed all pre-existing CCC-C or CCC-U motifs in the lacZ gene of pJC27 plasmid [53] into CCG-[C/U] to create a sequence that maintained the native amino-acid sequence but lacked CCC-[C/U] sequences by site-directed mutagenesis. To rule out the possibility of alternative initiation, we mutated the AUG at the third codon position of the original lacZ gene into AUC, resulting in a lacZ gene without any in-frame AUG in the first 100 codons except for the initiating codon. The modified lacZ gene was transferred to pKK223-3 and CCC-C (or CCC as a control) was inserted to codon position 5, 10, 20, 60 or 124 in the same CCC-C-ACC (or CCC-ACC for a control) context ( Fig. 1a ). In all cases, the correct lacZ product was synthesized only when tRNA Pro exhibited a +1FS movement at the CCC-C sequence. Note that the CAC codon following the CCC-C run in the 0-frame and the ACC codon following the CCC-C run in the +1-frame have frequencies of 1.1% and 2.4%, respectively, indicating similar supply levels of the corresponding tRNAs for expression of these alternative reading frames. To test the effect of a rare codon at the A-site, we made additional constructs where CCC at codon 124 was followed by in-frame CGG or UGG, the codon frequency of which was 0.5% and 1.4%, respectively. In these cases, the +1-frame codon is GGU with a usage frequency of 2.8%. Each CCC-C construct, as well as the control CCC construct, was introduced into the trmD - KO strain. A single colony was picked from an arabinose-containing Luria-Bertani (LB) plate and was grown in 3 ml LB without arabinose at 30 °C to OD 600 of 0.1 ( ∼ 3 h) to deplete pre-existing Trm5 in cells. Cultures were then inoculated into fresh LB with or without 0.2% (w/v) arabinose at a 50-fold dilution. The cultures with arabinose were harvested at OD 600 =0.4–0.6, whereas the cultures without arabinose were grown until they were slightly turbid. Cells were resuspended in Z buffer (10 mM KCl, 1 mM MgSO 4 , 50 mM β-mercaptoethanol, 60 mM Na 2 HPO 4 , 40 mM NaH 2 PO 4 , pH 7.0), permeabilized with 0.005% SDS and 10% chloroform, and the β-gal activity was measured [54] . The +1FS frequency was calculated as the ratio of the CCC-C reporter activity over the CCC reporter activity. Similar β-gal measurements for each CCC-C reporter versus the control CCC reporter were performed for E. coli efp − and efp + strains (JW4107-1 and BW25113 of the Yale E. coli Stock) grown and assayed at 30 °C. To complement the efp − strain, we introduced an EF-P-expressing plasmid by isolating the Nsi I- Spe I fragment (which co-expressed efp - yjeA - yjeK under the control of the T7 promoter) from the pST39 plasmid [23] and inserting it into pACYC184 at the Pst I and Xba I sites (which were created by mutagenesis), respectively. Expression of efp - yjeA - yjeK from the T7 promoter was enabled by lysogenization of E. coli efp − strain with λDE3 (Merck Millipore). The lysogenized cells harbouring a lacZ reporter construct were grown at 30 °C to OD=0.1–0.2, then 4–5 h in the presence of 0.1 mM IPTG to activate expression of the efp - yjeA - yjeK genes. Cells were then harvested and cell lysates assayed for β-gal at 30 °C. Growth assay for synthetic lethal phenotype To take advantage of a previously isolated isogenic pair of S. typhimurium wt-trmD and ts-trmD-S88L strains (GT7496 and GT7497, respectively, made by Dr G. Bjork), we introduced the efp-KO construct into this pair of strains. To do this, a kanamycin cassette was amplified from pKD4 by PCR with primers encompassing flanking regions of the efp gene: forward primer, 5′-GCGCCATTTTGTGGCTTAGCTACCAGTTAACAATTTCAGAGTGTAGGCTGGAGCTGCTTC-3′ and reverse primer, 5′-GGCGCAGCATACGCTGCACCATTTTTCCCGATAACGTAAAATGGGAATTAGCCATGGTCC-3′. Using the λ Red gene disruption method [52] , the PCR products were introduced into S. typhimurium wt-trmD and ts-trmD-S88L strains to obtain efp + and efp − strains in each. Cells from each strain were grown overnight at 30 °C in LB with chloramphenicol and kanamycin, and spotted by serial dilutions on LB plates with the same antibiotics and tested for growth at 30 or 44 °C. Pyrazinamidase assay The product of the pncA gene is nicotiamidase-pyrazinamidase (PZase), which catalyzes oxidation of pyrazinamide (PZA) into pyrazinoic acid (POA). Analysis of the enzymatic activity of PZase [55] was performed on cell lysates from the efp + and efp − strains, and the trmD - KO strain grown with or without 0.2% (w/v) arabinose. Cells were grown overnight in 200 ml LB media supplemented with antibiotics and 8 mM PZA at 30 °C. The cells were harvested and washed twice with 100 mM glycine, pH=6.0. Cells were then resuspended in 2 ml of glycine buffer, sonicated on ice and cell lysates collected by centrifugation at 16,000 g for 3 min at 4 °C. Protein concentration of the cleared lysates was determined by Bradford method. A lysate of 142 μl of each sample was mixed with 8 μl of 150 mM PZA (8 mM final) to start the reaction and aliquots were removed after incubation for 0’, 5’, 15’, 30’ and 60’ at 37 °C. The removed aliquots, which contained the product POA, were spun at 16,000 g for 5 min and a portion of the supernatant was mixed with 25 mM Fe(NH 4 ) 2 (SO 4 ) 2 to form a red-coloured complex for which OD 450 was measured. A standard curve was made by measuring OD 450 of a mixture of 25 mM Fe(NH 4 ) 2 (SO 4 ) 2 with increasing concentrations of POA. Specific activity was calculated at each time point as nmol of POA/min/mg protein. An E. coli XAC strain bearing the ts-trmD-S88L mutation [17] was also tested for this assay along with its parental strain ( wt - trmD ). Cell cultures were grown in 150 ml LB at 30 °C until the OD 600 reached 0.1 ( ∼ 3 h) and then split into two, with one growing at 30 °C and the other at 43 °C. The 30 °C culture was harvested when the OD 600 reached 0.4–0.6, whereas the 43 °C culture was harvested after 10 h when the intracellular TrmD activity was reduced to ∼ 10% of wild-type level [17] . How to cite this article: Gamper, H.B. et al. Maintenance of protein synthesis reading frame by EF-P and m 1 G37-tRNA. Nat. Commun. 6:7226 doi: 10.1038/ncomms8226 (2015).